Ouabain protects against adverse developmental programming of the kidney The kidney is extraordinarily sensitive to adverse fetal programming. Malnutrition, the most common form of developmental challenge, retards the formation of functional units, the nephrons. The resulting low nephron endowment increases susceptibility to renal injury and disease. Using explanted rat embryonic kidneys, we found that ouabain, the Na,K-ATPase ligand, triggers a calcium–nuclear factor-κB signal, which protects kidney development from adverse effects of malnutrition. To mimic malnutrition, kidneys were serum deprived for 24 h. This resulted in severe retardation of nephron formation and a robust increase in apoptosis. In ouabain-exposed kidneys, no adverse effects of serum deprivation were observed. Proof of principle that ouabain rescues development of embryonic kidneys exposed to malnutrition was obtained from studies on pregnant rats given a low-protein diet and treated with ouabain or vehicle throughout pregnancy. Thus, we have identified a survival signal and a feasible therapeutic tool to prevent adverse programming of kidney development. The mammalian kidney is a model organ for pattern formation. The formation of its functional units, the nephrons, depends on branching morphogenesis, mesenchymal–epithelial transition and inductive signalling [1] , [2] . The process of nephron formation is extraordinarily sensitive to the effects of adverse environmental events during certain critical windows of development. Fetal malnutrition, the most common form of developmental challenge, results in an irreversible reduction of nephrons [3] , [4] , [5] . In humans, the loss of nephrons caused by maternal low caloric intake or by placental insufficiency encompasses increased risk for renal disease and hypertension [6] , [7] . The ubiquitous integral plasma membrane protein, Na,K-ATPase, can, in addition to its well-studied function as an ion pump, function as a signal transducer [8] , [9] . Ouabain, a highly specific Na,K-ATPase ligand, tethers the catalytic α-subunit of Na,K-ATPase with the inositol 1,4,5-trisphosphate receptor (IP3R), and triggers the release of a series of calcium waves [10] , [11] , [12] , [13] . Calcium waves have emerged as a key regulator of early development [14] , [15] . However, little is known about the role of calcium in pattern formation and cell differentiation during later stages of embryonic life in mammals. Downstream effects of ouabain signalling include activation of the calcium-dependent transcription factor nuclear factor (NF)-κB and protection from apoptosis [16] . As those factors are implicated in developmental processes, we decided to study whether the signalling cascade triggered by ouabain might affect the developmental programming in kidneys exposed to malnutrition. To examine whether ouabain–calcium–NF-κB signalling might rescue the development of fetal kidneys exposed to malnutrition, we first used kidney explants from 14-day-old embryonic rats held in culture for 3 days. To mimic malnutrition, kidneys were serum deprived for 24 h. Imaging of intracellular calcium was performed in the outer cell layers of explanted kidneys. Spontaneous calcium waves were observed in the majority of cells, and both acute and chronic exposure to ouabain, in concentrations that had little or no effect on Na,K-ATPase pump function, were found to increase the number of calcium waves. As expected, serum-deprived kidneys displayed severe retardation of nephron formation and robust increase in apoptotic index (AI), but these effects were abolished if the kidneys were exposed to ouabain in concentrations that had no effect on intracellular sodium. To assess the role of the ouabain–calcium–NF-κB signalling pathway, we deprived the intracellular stores of calcium and blocked the transcriptional capacity of NF-κB. To obtain proof of principle that ouabain rescues the development of embryonic kidneys exposed to malnutrition, nephron endowment was examined in offspring of rat dams that had been given a low-protein diet and treated with ouabain or vehicle throughout pregnancy. Calcium activity in metanephric blastema cells To investigate whether spontaneous calcium activity can be observed at the time of nephron induction, we took advantage of the fact that branching morphogenesis occurs in the explanted kidney. Rat embryonic kidneys were removed at E14 and held in culture for 3 days. Imaging of intracellular calcium was performed in the outer cell layers of the kidney, consisting mainly of metanephric blastema cells in close contact with the epithelial ureteric bud, which triggers the epithelial conversion of blastema cells and the formation of primitive nephrons ( Fig. 1a,b ). Repetitive transient increases (waves) in intracellular calcium were observed in a majority of cells ( Fig. 1b–d and Supplementary Movie 1 ). These calcium waves could be attributed to the release of calcium from intracellular stores. Cyclopiazonic acid (CPA), a sarco-endoplasmic reticulum Ca 2+ -ATPase inhibitor, was used to deplete intracellular calcium stores. Application of the inhibitor caused, as expected, a temporary rise in intracellular calcium ( Fig. 1e ). Spontaneous calcium waves were rarely observed after the initial temporary rise. The role of extracellular calcium in the propagation of waves was investigated using blockers of voltage-gated calcium channels or by removal of calcium from the perfusion buffer. Notably, influx of calcium from the extracellular space seemed to be of little importance for the spontaneous calcium activity in the embryonic kidney ( Fig. 1f,g ). Calcium waves were still observed in cells exposed to calcium-free extracellular medium and endured in the presence of nifedipine, an inhibitor of voltage-gated calcium channels. This is, to the best of our knowledge, the first time that repetitive calcium waves have been observed in embryonic mammalian kidney. Repetitive calcium transients confer a unique precision and sensitivity on the activation of downstream target functions because of the numerous possibilities of temporal variations [17] . The current observations should offer new tools for studies and understanding of pattern formation and kidney development. 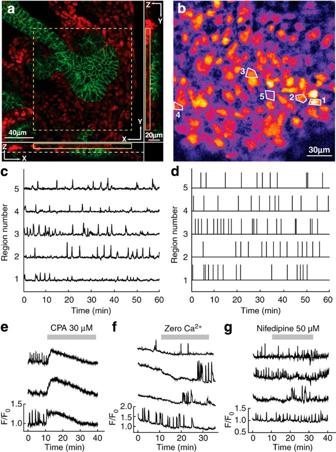Figure 1: Spontaneous calcium waves in embryonic rat kidney explants. (a) Orthogonal view of confocal images of embryonic kidney immunostained with Wt1 (red) and E-cadherin (green) antibodies to identify metanephric cells and ureteric bud cells, respectively. Note that the focal plane (dashed white line in the bottom image) is positioned beneath mesenchymal cells to visualize the underlying ureteric bud. (b) Pseudo-coloured confocal image of an embryonic kidney loaded with the calcium-sensitive dye Oregon Green BAPTA-1/AM (10 μM). Cells correspond to Wt1-labelled cells (red) within the selected region shown in panel a (yellow dashed region; yellow box, bottom and right image). (c) One hour recording of spontaneous calcium transients from regions 1–5 shown in panel b. Traces presented as normalized fluorescent intensity, F/F0. (d) Binary representation of calcium traces shown in panel c. Each vertical line corresponds to a calcium peak defined as 9% above background. (e) Application of 30 μM CPA caused a temporary rise in calcium, the calcium activity was negligible thereafter. (f) Kidneys were exposed to calcium-free extracellular solution, which did not affect the spontaneous activity during the observation period. (g) Spontaneous calcium transients were still observed after application of 50 μM nifedipine. Figure 1: Spontaneous calcium waves in embryonic rat kidney explants. ( a ) Orthogonal view of confocal images of embryonic kidney immunostained with Wt1 (red) and E-cadherin (green) antibodies to identify metanephric cells and ureteric bud cells, respectively. Note that the focal plane (dashed white line in the bottom image) is positioned beneath mesenchymal cells to visualize the underlying ureteric bud. ( b ) Pseudo-coloured confocal image of an embryonic kidney loaded with the calcium-sensitive dye Oregon Green BAPTA-1/AM (10 μM). Cells correspond to Wt1-labelled cells (red) within the selected region shown in panel a (yellow dashed region; yellow box, bottom and right image). ( c ) One hour recording of spontaneous calcium transients from regions 1–5 shown in panel b. Traces presented as normalized fluorescent intensity, F/F 0 . ( d ) Binary representation of calcium traces shown in panel c. Each vertical line corresponds to a calcium peak defined as 9% above background. ( e ) Application of 30 μM CPA caused a temporary rise in calcium, the calcium activity was negligible thereafter. ( f ) Kidneys were exposed to calcium-free extracellular solution, which did not affect the spontaneous activity during the observation period. ( g ) Spontaneous calcium transients were still observed after application of 50 μM nifedipine. Full size image Exposure to ouabain increases calcium activity Exposure of embryonic kidneys to ouabain caused a significant increase in the number of calcium waves ( Fig. 2a,b ). Kidneys were exposed to vehicle or 10 μM ouabain, a concentration that should activate the signalling function of Na,K-ATPase [16] but have little effect on the pump function ( Fig. 2e ). Recordings were taken for 26 min, and the number of calcium waves per cell was counted. We found a significant increase in the number of cells that displayed five or more waves during the recording in ouabain-treated kidneys ( Fig. 2b ). 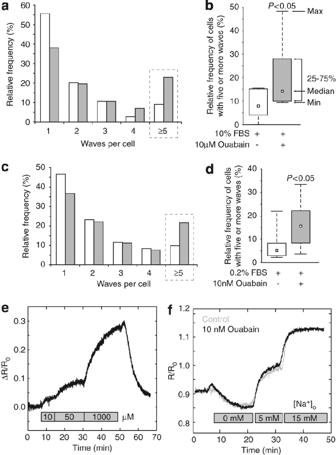Figure 2: Ouabain increases the number of spontaneous calcium waves. (a,b) Acute effect of ouabain. Kidneys were grown in standard serum conditions (10% FBS) and treated with vehicle (white bars) or 10 μM ouabain 1.5 h before and throughout the recording (grey bars). (a) Histogram of the number of waves per cell during the observation period of 26 min. (b) Box plot of the relative frequency of cells that displayed multiple (five or more) calcium waves during the observation period of 26 min. Statistical significance was estimated using the Mann–WhitneyU-test,P<0.05,z=−2.0831,n= 7 for vehicle-treated (white box) andn= 8 for ouabain-treated (grey box) kidneys. (c,d) Chronic effect of ouabain. The kidneys were serum deprived (0.2% FBS) and treated with vehicle (white bars) or 10 nM ouabain (grey bars) for the last 24 h of culture. (c) Histogram of the number of waves per cell during the observation period of 26 min. (d) Box plot of the relative frequency of cells that displayed multiple (five or more) calcium waves during the observation period of 26 min. Statistical significance was estimated using the Mann–WhitneyU-test,P<0.05,z=−2.506,n= 10 for vehicle-treated (white box) andn= 12 for ouabain-treated (grey box) kidneys. (e,f) Intracellular measurements of sodium in primary cultures of rat proximal tubule cells. (e) Ouabain dose–response. Cells were treated with different concentrations of ouabain. Graph shows the normalized 340/380 nm ratio, which increases as more sodium is accumulated in cells because of inhibition of Na,K-ATPase. Trace is an average from 15 cells. (f) Rat proximal tubule cells were treated with 10 nM ouabain or vehicle for 24 h. Three-point calibration using sodium ionophores was performed to measure the baseline sodium concentration (0–5 min). There were no differences between the initial sodium concentrations in ouabain-treated cells compared with cells treated with vehicle. Ouabain trace is an average of 20 cells. Control trace is an average of 40 cells. Figure 2: Ouabain increases the number of spontaneous calcium waves. ( a , b ) Acute effect of ouabain. Kidneys were grown in standard serum conditions (10% FBS) and treated with vehicle (white bars) or 10 μM ouabain 1.5 h before and throughout the recording (grey bars). ( a ) Histogram of the number of waves per cell during the observation period of 26 min. ( b ) Box plot of the relative frequency of cells that displayed multiple (five or more) calcium waves during the observation period of 26 min. Statistical significance was estimated using the Mann–Whitney U -test, P <0.05, z =−2.0831, n = 7 for vehicle-treated (white box) and n = 8 for ouabain-treated (grey box) kidneys. ( c , d ) Chronic effect of ouabain. The kidneys were serum deprived (0.2% FBS) and treated with vehicle (white bars) or 10 nM ouabain (grey bars) for the last 24 h of culture. ( c ) Histogram of the number of waves per cell during the observation period of 26 min. ( d ) Box plot of the relative frequency of cells that displayed multiple (five or more) calcium waves during the observation period of 26 min. Statistical significance was estimated using the Mann–Whitney U -test, P <0.05, z =−2.506, n = 10 for vehicle-treated (white box) and n = 12 for ouabain-treated (grey box) kidneys. ( e , f ) Intracellular measurements of sodium in primary cultures of rat proximal tubule cells. ( e ) Ouabain dose–response. Cells were treated with different concentrations of ouabain. Graph shows the normalized 340/380 nm ratio, which increases as more sodium is accumulated in cells because of inhibition of Na,K-ATPase. Trace is an average from 15 cells. ( f ) Rat proximal tubule cells were treated with 10 nM ouabain or vehicle for 24 h. Three-point calibration using sodium ionophores was performed to measure the baseline sodium concentration (0–5 min). There were no differences between the initial sodium concentrations in ouabain-treated cells compared with cells treated with vehicle. Ouabain trace is an average of 20 cells. Control trace is an average of 40 cells. Full size image We next examined the role of ouabain signalling in embryonic kidneys exposed to malnutrition. To mimic malnutrition, explanted kidneys were first cultured with standard serum (10% fetal bovine serum, FBS), and then starved by reducing the serum concentration to 0.2% and exposed either to vehicle or to 10 nM ouabain for 24 h. As the on-rate of ouabain binding exceeds the off-rate [18] , effective concentrations of ouabain can be considerably reduced (from 10 μM to 10 nM) when longer exposure times are used [13] . Spontaneous calcium activity was present in both groups of serum-deprived kidneys, but important quantitative differences were observed between ouabain and vehicle-exposed kidneys. In kidneys exposed to ouabain, significantly more cells displayed multiple calcium waves per unit time compared with kidneys not exposed to ouabain ( Fig. 2c,d ). Exposure to 10 nM ouabain for 24 h did not affect the intracellular sodium concentration ( Fig. 2f ). Ouabain inhibits cell death and increases proliferation The transcription factor NF-κB is a pleiotropic regulator of the inducible expression of many genes. Activation of NF-κB is a calcium-dependent process [19] . Activation of the Na,K-ATPase/IP3R signalling pathway by ouabain has been demonstrated to trigger nuclear translocation and activation of NF-κB. Here, we show that ouabain activates NF-κB in serum-deprived kidneys ( Fig. 3a ). NF-κB activates genes modulating apoptosis [20] and development, as well as responses of the immune system. Apoptosis was found to be a prominent feature in serum-deprived kidney explants ( Fig. 3b ). The AI was 7.0 ± 1.7% after serum deprivation for 24 h, whereas in kidneys exposed to normal serum for the entire culture period of 72 h, the AI was 1.9 ± 0.3%, which is in the range of that previously reported. It is important to note that the apoptotic effect was completely abolished if kidneys were exposed to ouabain during the time of serum deprivation (AI 1.2 ± 0.1%) ( Fig. 3b,c ). The antiapoptotic effect of ouabain required calcium release from intracellular stores. Thus, when serum-deprived kidneys were incubated with both ouabain and CPA, the AI was no longer different from that observed in vehicle-treated kidneys. CPA alone had no effect on the AI. To assess the link between ouabain-dependent NF-κB activation and protection from apoptosis in the embryonic kidney, we used helenalin, an NF-κB inhibitor. Helenalin abolished the antiapoptotic effect of ouabain, but had no effect on apoptosis on its own ( Fig. 3c ). 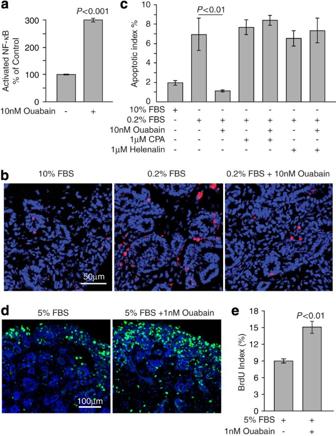Figure 3: Ouabain protects from apoptosis in malnourished kidneys through the Na,K-ATPase/IP3R/NF-κB signalling pathway. (a) Ouabain increased NF-κB abundance in the nucleus. NF-κB p65 Trans-aminase assay was used to detect translocation of NF-κB to the nucleus. Values are mean ± s.e.m.;P<0.001,n= 3. (b) Representative confocal images of embryonic kidneys labelled with terminal deoxynucleotidyl transferase-mediated dUTP nick-end labelling (TUNEL, red) to detect apoptotic cells and 4′,6-diamidino-2-phenylindole (DAPI, blue) to detect nuclei. (c) Ouabain reduced serum deprivation-triggered apoptosis in kidneys. AI was given as % of apoptotic cells. AI was determined by analysing 3–4 randomly selected areas, with 1,000–2,000 cells in each area, from three independent experiments. A volume of 1 μM CPA or 1 μM helenalin abolished the antiapoptotic effect of ouabain. Values are mean ± s.e.m.,P<0.01,n= 3. (d) Embryonic kidneys labelled with BrdU (5-bromodeoxyuridine, green) and DAPI (blue) to detect proliferating cells and cell nuclei, respectively. (e) Ouabain significantly stimulated cell proliferation. BrdU index was given as % of BrdU-positive cells. In each preparation, 5–7 randomly selected areas were examined and in each area around 1,000 DAPI-stained cells were counted. Values are mean ± s.e.m.,P<0.01,n= 3. Figure 3: Ouabain protects from apoptosis in malnourished kidneys through the Na,K-ATPase/IP3R/NF-κB signalling pathway. ( a ) Ouabain increased NF-κB abundance in the nucleus. NF-κB p65 Trans-aminase assay was used to detect translocation of NF-κB to the nucleus. Values are mean ± s.e.m. ; P <0.001, n = 3. ( b ) Representative confocal images of embryonic kidneys labelled with terminal deoxynucleotidyl transferase-mediated dUTP nick-end labelling (TUNEL, red) to detect apoptotic cells and 4′,6-diamidino-2-phenylindole (DAPI, blue) to detect nuclei. ( c ) Ouabain reduced serum deprivation-triggered apoptosis in kidneys. AI was given as % of apoptotic cells. AI was determined by analysing 3–4 randomly selected areas, with 1,000–2,000 cells in each area, from three independent experiments. A volume of 1 μM CPA or 1 μM helenalin abolished the antiapoptotic effect of ouabain. Values are mean ± s.e.m., P <0.01, n = 3. ( d ) Embryonic kidneys labelled with BrdU (5-bromodeoxyuridine, green) and DAPI (blue) to detect proliferating cells and cell nuclei, respectively. ( e ) Ouabain significantly stimulated cell proliferation. BrdU index was given as % of BrdU-positive cells. In each preparation, 5–7 randomly selected areas were examined and in each area around 1,000 DAPI-stained cells were counted. Values are mean ± s.e.m., P <0.01, n = 3. Full size image Low concentrations of ouabain, which do not perturb the resting cellular ionic milieu, can stimulate cell proliferation [21] . In rat embryonic kidney explants, the majority of proliferating cells are observed in metanephric blastema cells. Ouabain signalling was found to enhance cell proliferation in these cells to approximately 15% ( Fig. 3d,e ). Ouabain increases expression of NF-κB target genes The molecular mechanisms by which NF-κB protects from apoptosis in the embryonic kidney are not well understood. They may involve enhanced activation of Wt1 and Pax2 , which belong to the large number of well-characterized genes that have been identified to have a crucial role in pattern formation and differentiation of the embryonic kidney. Both genes are activated by calcium signalling pathways and NF-κB [22] , [23] . The expression of Wt1 and Pax2 mRNA was similar in serum-exposed and serum-deprived kidneys ( Fig. 4a,b ). In contrast, serum-deprived kidneys that had been exposed to ouabain had increased expression levels of Wt1 and Pax2 mRNA ( Fig. 4a,b ). These results imply that exposure to malnutrition did not have a direct effect on Na,K-ATPase/IP3R signalling, but that the enhancement of this signal by treatment with exogenous ouabain could function to compensate for the loss of other, so far not identified, factors. The ouabain effects on Wt1 and Pax2 mRNA were abolished in kidneys simultaneously exposed to ouabain and helenalin ( Fig. 4c,d ). 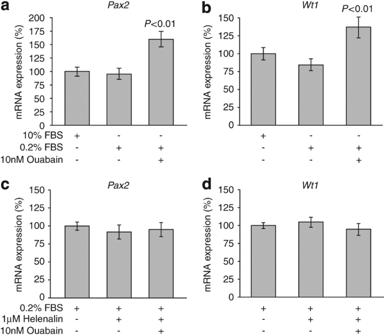Figure 4: Ouabain increases expression ofWt1andPax2. (a,b) Expression ofPax2mRNA (a) andWt1mRNA (b) in kidneys cultured on filters with or without ouabain, relative to control (10% FBS),n= 7;Pax2,P<0.01;Wt1,P<0.01. (c,d) Expression ofPax2(c) andWt1(d) in kidney explants treated with 1 μM helenalin alone or combined with ouabain, relative to control (0.2% FBS). Helenalin treatment abolished the increased expression of both genes observed after ouabain treatment,n= 7. Values are mean ± s.e.m. Figure 4: Ouabain increases expression of Wt1 and Pax2 . ( a , b ) Expression of Pax2 mRNA ( a ) and Wt1 mRNA ( b ) in kidneys cultured on filters with or without ouabain, relative to control (10% FBS), n = 7; Pax2 , P <0.01; Wt1 , P <0.01. ( c , d ) Expression of Pax2 ( c ) and Wt1 ( d ) in kidney explants treated with 1 μM helenalin alone or combined with ouabain, relative to control (0.2% FBS). Helenalin treatment abolished the increased expression of both genes observed after ouabain treatment, n = 7. Values are mean ± s.e.m. Full size image Ouabain rescues nephron formation ex vivo and in vivo As fetal malnutrition is associated with enhanced renal apoptosis and decreased rate of cell proliferation [24] , we next sought to determine whether ouabain may protect from the effects of malnutrition on nephron endowment. E14 kidneys were either cultured under standard serum conditions (10% FBS) for the entire culture period, or serum starved (0.2% FBS) during the last 24 h of culture in the presence or absence of 10 nM ouabain. Kidneys were subsequently stained with markers for glomeruli and branching tubules ( Fig. 5a ). Serum deprivation caused a profound decrease in the number of glomeruli, but exposure to ouabain almost completely prevented this effect ( Fig. 5b ). The rescuing effect of ouabain required the release of calcium from the intracellular stores, as well as activation of NF-κB ( Supplementary Fig. S1 ). Ureteric branching was also retarded by serum deprivation but rescued by exposure to ouabain ( Supplementary Fig. S1 ). 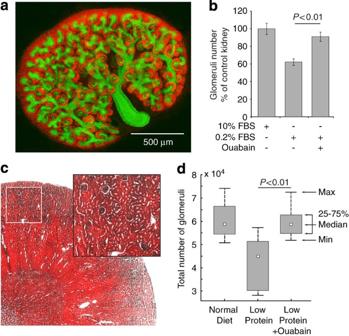Figure 5: Ouabain rescues nephrogenesis in fetal malnutrition. (a) Representative confocal image of kidney stained withWt1(red) and E-cadherin (green) antibodies to identify newly formed glomeruli and ureteric branches. (b) Serum deprivation in embryonic kidney explants (n= 15) decreased the number of glomeruli by 38 ± 4%, compared with kidneys grown in 10% FBS (n= 9). In serum-deprived kidneys treated with ouabain (n= 14), the number of glomeruli was not significantly different than in kidneys grown in 10% FBS. Values are mean ± s.e.m.P<0.01. (c) Representative image of haematoxylin- and eosin-stained kidney used for the stereological examination of total glomeruli number. (d) Total number of glomeruli in 4-week-old rats exposed to a normal protein diet or a low-protein diet with or without ouabain during fetal life. Diagram shows total number of glomeruli per kidney. The total number of glomeruli per kidney, in rats exposed to low protein, was significantly reduced. Ouabain rescued the effect of a low-protein diet with regard to glomeruli formation. The number of glomeruli in the low protein/ouabain-treated group was not different from the number of glomeruli in the control group. Statistical significance was estimated using a two-tailedU-test,P<0.01,z=2.836.n= 8 kidneys/group. Figure 5: Ouabain rescues nephrogenesis in fetal malnutrition. ( a ) Representative confocal image of kidney stained with Wt1 (red) and E-cadherin (green) antibodies to identify newly formed glomeruli and ureteric branches. ( b ) Serum deprivation in embryonic kidney explants ( n = 15) decreased the number of glomeruli by 38 ± 4%, compared with kidneys grown in 10% FBS ( n = 9). In serum-deprived kidneys treated with ouabain ( n = 14), the number of glomeruli was not significantly different than in kidneys grown in 10% FBS. Values are mean ± s.e.m. P <0.01. ( c ) Representative image of haematoxylin- and eosin-stained kidney used for the stereological examination of total glomeruli number. ( d ) Total number of glomeruli in 4-week-old rats exposed to a normal protein diet or a low-protein diet with or without ouabain during fetal life. Diagram shows total number of glomeruli per kidney. The total number of glomeruli per kidney, in rats exposed to low protein, was significantly reduced. Ouabain rescued the effect of a low-protein diet with regard to glomeruli formation. The number of glomeruli in the low protein/ouabain-treated group was not different from the number of glomeruli in the control group. Statistical significance was estimated using a two-tailed U -test, P <0.01, z =2.836. n = 8 kidneys/group. Full size image The studies conducted on kidney explants collectively indicate that ouabain protects from the adverse effects of malnutrition on kidney development. To test this concept in vivo , pregnant rats were given a low-protein diet. Minipumps delivering either ouabain or vehicle were implanted subcutaneously during the second day of pregnancy. Pregnant rats receiving a normal protein diet served as control. The offspring of all groups were killed at the age of 4 weeks and kidneys were processed for stereological examination of glomeruli number. In rats, formation of glomeruli is completed at 1 week of age. Consistent with reports from other investigators [24] , [25] , we found a highly significant reduction in the number of glomeruli in the low-protein group as compared with the normal protein group. It is important to note that this reduction was abolished in the offspring of low protein-diet-fed mothers that had been exposed to ouabain during pregnancy ( Fig. 5c,d ). In this study, we present a feasible principle for prevention of adverse fetal programming. The concept of fetal programming has emerged from a large number of human epidemiological and animal experimental studies, demonstrating a link between adverse exposures during fetal life and adult-onset diseases [26] , [27] . The kidney is extraordinarily sensitive to the effects of an adverse environment during critical windows of development. We have used the kidney as a model organ to test whether ouabain-triggered calcium–NF-κB signalling may rescue from the effects of adverse developmental programming. Ouabain-triggered calcium release is mediated by direct interaction between Na,K-ATPase and the IP3R [9] , [13] . As these ubiquitous proteins are expressed from the very first developmental stage, and as the role of calcium [1] and NF-κB [28] , [29] signalling during development is well documented, we hypothesized that the Na,K-ATPase/IP3R signalosome might have a protective effect during development. The effects that Na,K-ATPase/IP3R signalling will have on normal development remain to be elucidated. Several lines of evidence suggest that ouabain is a mammalian hormone produced in the adrenals and hypothalamus [30] , and that circulating levels of ouabain are high during pregnancy [31] . Ouabain functions by stabilizing Na,K-ATPase in one conformation. It is possible that, during development, alterations in the conformational equilibrium of Na,K-ATPase, which would favour an interaction with the IP3R, might occur even in the absence of a ligand. Our results have important medical and socio-economical consequences. Experimental models have unequivocally shown that fetal malnutrition, caused by maternal calorie restriction or placental insufficiency, leads to offspring with fewer glomeruli. Similarly, it has been unequivocally shown that low nephron endowment has an adverse effect on the outcome of all kidney diseases and is a major risk factor for chronic renal disease [3] , [6] , [7] , [25] , [32] . Studies on autopsy material have confirmed that low birth weight, a hallmark of fetal growth restriction, is associated with reduced number of nephrons in humans [33] , [34] . A recent large cohort study, comprising data on all births in Norway between 1967 and 2004, showed that low birth weight was associated with a 70% increased risk for end-stage renal failure [35] . Chronic kidney diseases represent a major socioeconomical burden, both in industrial and developing countries. For example, there are now more than 20 million Americans who have some evidence of chronic kidney disease and are at risk of developing kidney failure, and the annual costs to treat kidney disease in the United States are more than one quarter (27.6%) of Medicare's expenditures [36] . Cardiovascular and renal disease risks are entwined through hormonal mechanisms, and chronic kidney diseases are associated with increased risk for hypertension and death in cardiovascular disease. Yet, despite overwhelming evidence that fetal malnutrition endangers kidney development and results in an irreversible loss of nephrons and increased risk for renal disease and hypertension, there is, as yet, no drug available that would alleviate the effects of fetal malnutrition on nephron formation. Results from this study imply that ouabain, or analogues of ouabain, can efficiently be used for this purpose. Organ culture Animal experiments were approved by the Institutional Animal Care and Use Committee of the Karolinska Institutet. Embryonic methanephroi were isolated from E14 Sprague–Dawley rat embryos, and cultured on a Transwell filter (0.4-μm pore size, CoStar) within individual wells of a 12-well tissue culture dish containing 800 μl of Dulbecco's modified Eagle's medium/F12 media (Invitrogen) supplemented with 10% FBS. The kidneys were cultured at 37 °C in an air atmosphere containing 5% CO 2 and 100% humidity for a total of 72 h. To starve kidneys, 0.2% FBS was used during the last 24 h of culture. Calcium imaging Kidneys were loaded 50–80 min before recording with the calcium-sensitive dye Oregon Green BAPTA-1/AM (10 μM, Molecular Probes), and perfused with Krebs Ringer Buffer, consisting of, in mM, 100 NaCl, 4 KCl, 20 HEPES, 25 NaHCO 3 , 1 CaCl 2 , 1.2 MgCl 2 , 1 NaH 2 PO 4 ·H 2 O, 10 D -glucose, pH 7.35, at 37 °C. In one protocol, CaCl 2 was excluded and replaced with 250 μM ethylene glycol bis(β-aminoethylether)- N,N,N ′, N ′,-tetraacetic acid ( Fig. 1f ). Intracellular calcium was imaged at 0.5 Hz using an argon laser (488 nm) and LP505 long-pass filter on a LSM 510 Zeiss Duo inverted microscope. Image analysis was performed using ImageJ ( http://rsbweb.nih.gov/ij/ ) and custom-made scripts in MATLAB (The MathWorks). Each calcium trace was normalized using median filtered baseline fluorescence. Low amplitude and high frequency noise were removed from the normalized signal using wavelet transformations (Daubechies 3-d order). In the normalized and filtered data, a wave was defined as a signal that is 9% over baseline [37] . In vitro model Whole-mount immunostaining of kidney explants was used to quantify the number of glomeruli and ureteric buds. Anti-E-cadherin (mouse, 1:500 dilution, BD Bioscience) and anti- Wt1 (rabbit, 1:200, Santa Cruz) were used to detect ureteric branches and glomeruli, respectively. Alexa 488 antimouse (1:200, Molecular Probes) and Alexa 546 antirabbit (1:400, Molecular Probes) were used as secondary antibodies. Glomeruli and ureteric terminal tips were counted in the largest sagittal cross-section from each kidney. The number of glomeruli and ureteric terminal tips per maximal cross-section was taken as an index of total kidney glomeruli and ureteric tip numbers [38] . Results are given as the percentage of the number of glomeruli and ureteric branches observed in the control kidney, which is exposed to standard serum (10% FBS) during the entire culture period. AI was determined using the 'ApopTag Red In Situ Apoptosis Detection kit' (Chemicon) according to the protocol for cryosectioned samples. Bromo-deoxi-uridine, BrdU, incorporation was used to estimate cell proliferation. The cell proliferation kit (RPN20, Amersham Biosciences) was used according to the manufacturer's recommendations for cryopreserved and cryosectioned samples. NF-κB activity was measured by The TransAM NFκB p65 Kit (Active Motif) according to the manufacturer's recommendations. Three to four kidneys grown on the same filter were used for nuclear extraction for each sample. Ouabain treatment Rat kidney cells are known to predominantly express the Na,K-ATPase α1 isoform. This isoform is, in rodents, much less sensitive to ouabain than the α2 and α3-isoforms. Supplementary Figure S2 shows that the embryonic kidneys we studied only express the α1-isoform. The ouabain concentration required for signal activation is lower than that required for inhibition of ion transport [13] , [16] . Here, we show that acute exposure to 10 μM ouabain, which is the concentration we use for acute treatments, has a negligible effect on intracellular sodium concentration ( Fig. 2e ). As the on-rate of ouabain exceeds the off-rate [18] , effective concentrations of ouabain can be considerably reduced when longer exposure times are used. A volume of 10 nM ouabain was added to the culture medium during the last 24 h of culture. A 24 h exposure of rat renal cells to 10 nM ouabain had no effect on intracellular sodium concentration ( Fig. 2f ). In the proliferation protocol ( Fig. 3d,e ), we observed significant effects using 1 nM ouabain. Intracellular sodium measurements Primary cultures of rat proximal tubule cells were prepared as described previously [10] , [39] , [40] . The cells were loaded with 10 μM SBFI-AM (Invitrogen) for 45 min at room temperature, followed by washing and 30 min de-esterification in normal media with 1 mM Probenecid (Invitrogen) at 37 °C. Sodium measurements were taken at 35 °C in a closed chamber (FCS3, Bioptechs) with a cooled CCD camera (ORCA-ERG, Hamamatsu) mounted on an upright microscope (Axioskop 2 FS, Zeiss) with a Zeiss Fluar 40 × 1.3 NA oil objective. Excitation at 340 and 380 nm was performed with a monochromator (Polychrome IV, TILL Photonics). Data acquisition and analysis was performed using MetaFluor (Molecular Devices). Cells were superfused with Krebs-Ringer with 1 mM probenecid. Calibration was performed using perfusion buffer with [Na + ]+[K + ]+[Choline + ]=140 and [Na + ]=0, 5 or 15 mM, with 6 μM Gramicidin D, 20 μM Monensin and 1 mM Ouabain (all from Sigma). Expression of Wt1 and Pax2 genes Total RNA was extracted from a single embryonic kidney using the Aurum Total RNA Mini Kit (Bio-Rad) according to the manufacturer's recommendations. Relative real-time reverse transcription–PCR was performed according to the manufacturer's recommendations for iScript One-Step RT–PCR Kit with SYBR Green (Bio-Rad). Quantification was performed in quadruplet for each sample. Commercial 18S Classic II primers (Ambion) were used to control genomic DNA contamination, to normalize RNA quality and starting quantity, as well as random tube-to-tube variation in reverse transcription (RT) and PCR reactions. Serial dilution of reference RNA sample as template was used to generate standard curve for each real-time RT–PCR experiment. The standard curve was constructed by plotting the log of the starting quantity of total RNA against the C t value. The starting quantity of Wt1 and Pax2 mRNA in each test sample was estimated using iQ iCycler software (Bio-Rad) using values from the standard curve and normalized using 18S RNA as reference. Values are presented as % of control (10% FBS in Figure 4a,b , 0.2% FBS in Figure 4c,d ). Rat Wt1 mRNA structure [41] (accession number X69716 ) was used to select Wt1 -specific primers: upper, 5′-TGCCACACCCCTACCGACAGTT-3′; lower, 5′-CTTCAAGGTAGCTCCGAGGTTCATC-3′. The position of rat Wt1 primers corresponds to a common part of all Wt1 mRNA splice variants. The rat Pax2 mRNA structure [42] (accession number XM_239083.4 ) was used to select Pax2 -specific primers: upper, 5′-TACACTGATCCTGCCCACATTAGA-3′; lower, 5′-GGATAGGAAGGACGCTCAAAGACT-3′. The rat Pax2 PCR fragment corresponds to human Pax2 mRNA splice variants A and E (accession numbers NM_003987 and NM_003990 , respectively). In vivo study Pregnant Sprague–Dawley rats (Scanbur AB) were given either a low (9%) or a normal (18%) protein diet (Special Diets Services) immediately after mating. Under Isofluran anaesthesia, osmotic pumps (Alzet Osmotic Pumps), delivering either ouabain dissolved in PBS (15 μg ouabain per kg body weight per day) or vehicle, were implanted subcutaneously on the second day of pregnancy. This daily dose of ouabain has previously been shown to result in plasma levels of ouabain around 1 nM [43] and to have little side effects, except a slight increase in systolic (but not diastolic) pressure [44] . The offspring of the three groups were killed at the age of 4 weeks and their kidneys were processed for stereological examination of glomerular number. The gender distribution was similar in all groups. Paraffin-embedded kidneys were serially sectioned (10–20 μm slices) and stained with haematoxylin and eosin. High-resolution images were recorded using a 5 × 0.16 NA objective and a motorized stage to cover the full area of each section. Images were automatically stitched together for a field of view of 15×15 mm. The contrast of each image was adjusted to maximize detection of glomeruli. Stereological analysis was performed using a modified form of the disector method. The disector method is based on the analysis of image pairs, images taken of sections in direct succession, and identification of unique objects [25] . The density of glomeruli was calculated as the number of unique glomeruli divided by the volume of the slice. Kidneys were weighed immediately after dissection and kidney volume was calculated from the volume/weight ratio 1.040 [25] . Total number of glomeruli per kidney was calculated as density multiplied by volume. Statistical analysis Statistical significance of the stereological counting of the total number of glomeruli per kidney, the acute effect of ouabain and chronic exposure to low doses of ouabain on calcium activity and the results of the in vivo experiments were estimated by the nonparametric Mann–Whitney U -test (two-tailed, P <0.05). For other data, one-way analysis of variance was applied ( P <0.05). How to cite this article: Li, J. et al . Ouabain protects against adverse developmental programming of the kidney. Nat. Commun. 1:42 doi: 10.1038/ncomms1043 (2010).